A prevalent cancer susceptibility APOBEC3A hybrid allele bearing APOBEC3B 3′UTR enhances chromosomal DNA damage Human APOBEC3A (A3A) cytidine deaminase is a host enzyme that can introduce mutations into chromosomal DNA. As APOBEC3B (A3B) encodes a C-terminal catalytic domain ~91% identical to A3A, we examined its genotoxic potential as well as that of a highly prevalent chimaeric A3A–A3B deletion allele (Δ A3B ), which is linked to a higher odds ratio of developing breast, ovarian and liver cancer. Interestingly, breast cancer genomes from Δ A3B −/− patients show a higher overall mutation burden. Here it is shown that germline A3B can hypermutate nuclear DNA, albeit less efficiently than A3A. Chimaeric A3A mRNA resulting from Δ A3B was more stable, resulting in higher intracellular A3A levels and greater DNA damage. The cancer burden implied by the higher A3A levels could be considerable given the high penetration of the Δ A3B allele in South East Asia. The human seven gene APOBEC3 (A3) cluster locus encodes six functional polynucleotide cytidine deaminases (A3A–C and A3F–H) some of which are involved in cellular defence against viruses and retroelements through cytidine deamination of single-stranded DNA (ssDNA) [1] . A3A notably is able to hypermutate nuclear DNA (nuDNA) resulting in the formation of double-stranded DNA breaks (DSBs) and apoptosis [2] , [3] , [4] . In addition, A3A could deaminate DNA molecules harbouring a variety of 5-oxidized cytidine bases including 5-methylcytidine (5Me-dC; refs 5 , 6 , 7 ). These findings parallel the accumulation of cancer genome sequences that revealed far more somatic mutations per genome than hitherto imagined, the majority being, with notable exceptions, GC→AT transitions [8] , [9] , [10] , [11] . In view of the above and the hallmark 5′TpC editing signature associated with cytidine deamination, it is now accepted that A3 molecules are involved in the genesis of cancer genomes [9] , [12] , [13] , [14] . A3A and the C-terminal domain of A3B differ by 9% at the amino-acid level. A3B has been clearly shown to edit viral genomes such as human immunodeficiency virus (HIV) [15] , human T-lymphotrophic virus [16] , [17] and hepatitis B virus (HBV) [18] , [19] . Two recent reports suggested A3B editing of nuDNA [20] , [21] . However, the degree of editing, of the order of a few mutations per kilobase, was unlike that observed for A3A (hundreds per kilobase), and probably represents PCR background [22] . The role of A3B in genome editing is intriguing, given that deletion of most of the A3B gene results in a higher odds ratio of developing breast, ovarian or liver cancer [23] , [24] , [25] , [26] . Indeed, complete genome sequencing of Δ A3B −/− breast cancer genomes revealed a higher than average mutation burden greatly consolidating these genetic studies [27] . The 29.5-kb deletion leaves a chimaeric A3A–A3B transcript that does not affect the A3A protein sequence but terminates with the A3B 3′ untranslated region (UTR). Yet it is contra-intuitive that deletion of a nuDNA mutator enzyme increases the risk of cancer, especially as there was a heterozygous effect suggesting a gene-dosage effect. As this is a highly prevalent polymorphism with frequencies ~30–40% in South East Asia and China, and >90% in Oceania [28] , understanding the underlying mechanism is of concern. It turns out that while both A3A and A3B can generate mutations in nuDNA, A3A alone is capable of inducing detectable DSBs. Moreover, it transpires that the A3A–A3B deletion polymorphism results in increased chimaeric A3A mRNA and protein levels that translate into more DNA damage. This may underlie an increased cancer predisposition of individuals harbouring this allele. Functional attenuation of APOBEC3B in Escherichia coli The starting point was the observation that human A3B cDNA expression plasmids could occasionally accumulate somatic mutations. Our original A3B construct derived from an Image clone encoding a known but minor T146K polymorphism (A3Bwh) [4] had recently acquired two somatic mutations, notably F308L and W359L ( Fig. 1a ). Another available plasmid, A3Blan (ref. [29] ), encoded eight amino-acid substitutions, K62E, L80P, F107L, T146K, M193V, D205G, T337A and R372K, whereas A3Btok (refs 21 , 30 ) encoded the T146K polymorphism ( Fig. 1a ). As none of the other mutations are known polymorphisms, they were probably selected to attenuate toxic A3B expression via leaky T7 promoters in E. coli, as has been reported for some A3 constructs [31] , [32] . V5-tagged versions of germline A3B and A3Btok proved to be genetically unstable while A3Blan posed no problem. To overcome this issue, a germline A3B cDNA retaining the entire intron 7 was synthetized and cloned into pcDNA3.1 (plasmid pA3Bi7). This nontoxic and stable construct was subsequently used to generate A3B derivatives, notably the T146K polymorphism, an E255Q null mutant as well as individual mutations F308L and W359L found in A3Bwh. Western blot analysis confirmed that A3B proteins were produced in comparable amounts ( Fig. 1b ), all of them exhibiting A3B classical nuclear localization ( Supplementary Fig. 1a ). 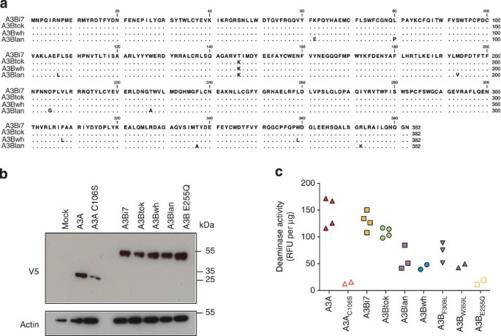Figure 1: A3B molecular clones and cytidine deamination activity. (a) ClustalW alignment of A3B proteins. Only variable residues are shown. (b) Representative western blot analysis from three independent experiments of V5-tagged A3B in human HEK 293T-UGI cells. β-Actin was used as loading control. (c)In vitrodeamination assay performed on TAMRA–FAM-coupled oligonucleotide using transfected 293T lysates from two experiments performed in duplicates. Background fluorescence obtained with mock-transfected cells was subtracted, and A3A A3AC106Sand A3BE255Qcatalytic mutants were used as a negative control. RFU, Relative Fluorescence Unit. Figure 1: A3B molecular clones and cytidine deamination activity. ( a ) ClustalW alignment of A3B proteins. Only variable residues are shown. ( b ) Representative western blot analysis from three independent experiments of V5-tagged A3B in human HEK 293T-UGI cells. β-Actin was used as loading control. ( c ) In vitro deamination assay performed on TAMRA–FAM-coupled oligonucleotide using transfected 293T lysates from two experiments performed in duplicates. Background fluorescence obtained with mock-transfected cells was subtracted, and A3A A3A C106S and A3B E255Q catalytic mutants were used as a negative control. RFU, Relative Fluorescence Unit. Full size image A3B plasmids were transfected into 293T cells and cellular lysates were used in a fluorescence resonance energy transfer based in vitro deamination assay where C to U conversion in a TAMRA-FAM-labelled DNA oligonucleotide allows fluorescence detection following cleavage by uracil-DNA glycosylase (UNG) activity [31] , [33] . All A3B constructs showed cytidine deamination activity, whereas A3A C106S and A3B E255Q null mutants did not ( Fig. 1c ). If A3Bi7 and A3Btok displayed cytidine deaminase activity comparable to A3A, A3Bwh and A3Blan showed diminished activity, whereas F308L and W359L individually showed attenuated activity. Turning to cell-based systems, A3 activity was assessed by HBV genome editing that has proven to be the most sensitive in vivo assay for A3 activity [19] , [34] . Following co-transfection of A3 plasmids along with the pCayw HBV infectious molecular clone, total cellular DNA was extracted and HBV editing was analysed by differential DNA denaturation PCR (3DPCR), a technique that allows recovery of AT rich DNA [35] . For all A3B constructs, HBV DNA was recovered at temperatures below the limiting denaturation temperature Td=89.0 °C for unedited DNA obtained with inactive A3B E255Q , A3A C106S mutants or mock-transfected cells ( Supplementary Fig. 1b ). While A3Bi7 and A3Btok transfections allowed recovery of edited HBV DNA down to 81.3 °C, again A3Blan and A3Bwh were less active, DNA being recovered at higher Tds. Once again F308L and W359L proved to be attenuating mutations ( Supplementary Fig. 1b ). APOBEC3B can deaminate nuDNA and 5-methylcytidine The ability of A3Bi7 to edit nuDNA and 5Me-dC, hallmark activities of A3A, was investigated. A3B plasmids were transfected into 293T-UGI (uracil-DNA glycosylase inhibitor) cells, which stably express the UNG inhibitor UGI [33] , allowing detection of nuDNA editing as in the case of A3A (ref. 4 ). Edited TP53 nuDNA was recovered using 3DPCR from A3Bi7 and A3Btok transfections ( Fig. 2a ). Sequences were peppered with C to T mutations preferentially on the minus strand ( Fig. 2b,c ), reflecting an A3 deamination process occurring on the non-transcribed template strand [36] . Dinucleotide analysis of edited bases showed a strong 5′TpC preference for cytidine deamination ( Fig. 2d ). By contrast A3Bwh and A3Blan failed to edit nuDNA ( Fig. 2a ). Once again, F308L and W359L both abrogated nuDNA editing ( Fig. 2a ). To confirm this in another cell type, we co-transfected QT6 cells, which are devoid of any APOBEC editing background, with A3B plasmids along with a UGI-coding plasmid. 3DPCR amplification of a segment of quail CMYC recovered hyperedited sequences with C→T transitions in the 5′TpC dinucleotide context for A3Bi7 and A3Btok constructs to 89.6 °C and 88.7 °C respectively, below the restrictive temperature Td=91.7 °C obtained for controls ( Supplementary Fig. 2a–c ). 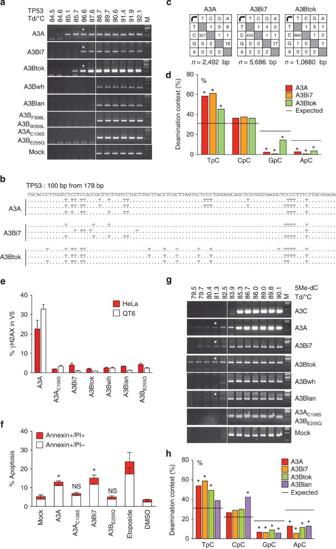Figure 2: A3B mutator enzymes and nuDNA damage. (a) TP53-specific 3DPCR gels after 293T-UGI transfections with A3 proteins. Asterisks denote samples that were cloned and sequenced. (b) Selection of hypermutated TP53 sequences after A3 transfection in 293T-UGI cells. (c) Mutation matrices of hyperedited sequences on TP53 minus strand DNA. The numbers below the matrices indicate the number of bases sequenced. (d) 5′ Dinucleotide analysis of the deamination context performed on minus strand DNA. *Significant deviation from expected values (χ2-test,P<0.05,n=35 for A3A,n=64 for A3Bi7,n=65 forA3Btok). (e) Fluorescence-activated cell sorting (FACS) analysis of γH2AX-positive HeLa and QT6 cells gated on V5-positive cells after A3 transfection at 48 h. Error bars represent s.d. from six independent transfections. (f) FACS analysis of early apoptosis (Annexin V-positive, PI-negative cells—white) and late apoptosis/necrosis (Annexin V-positive, PI double-positive cells—red) 36 h post transfection. Differences compared with mock-transfected cells were calculated using the Mann–Whitney test (*P<0.05). Error bars represent s.d. from four independent transfections. Top error bars relate to Annexin staining, whereas lower error bars represent s.d. for PI staining among Annexin+ cells. DMSO, dimethylsulfoxide; NS, not significant. (g) 3DPCR gels after QT6 transfections with A3 constructs along with 5Me-dC-substituted HIV-1envgene matrix. Asterisks denote the samples that were cloned and sequenced. (h) 5′ Dinucleotide analysis of the deamination context performed on minus strand DNA. *Significant deviation from expected values (χ2-test,P<0.05,n=25 for A3A,n=29 for A3Bi7,n=14 forA3Btok,n=21 for A3Blan). Figure 2: A3B mutator enzymes and nuDNA damage. ( a ) TP53-specific 3DPCR gels after 293T-UGI transfections with A3 proteins. Asterisks denote samples that were cloned and sequenced. ( b ) Selection of hypermutated TP53 sequences after A3 transfection in 293T-UGI cells. ( c ) Mutation matrices of hyperedited sequences on TP53 minus strand DNA. The numbers below the matrices indicate the number of bases sequenced. ( d ) 5′ Dinucleotide analysis of the deamination context performed on minus strand DNA. *Significant deviation from expected values ( χ 2 -test, P <0.05, n =35 for A3A, n =64 for A3Bi7, n =65 forA3Btok). ( e ) Fluorescence-activated cell sorting (FACS) analysis of γH2AX-positive HeLa and QT6 cells gated on V5-positive cells after A3 transfection at 48 h. Error bars represent s.d. from six independent transfections. ( f ) FACS analysis of early apoptosis (Annexin V-positive, PI-negative cells—white) and late apoptosis/necrosis (Annexin V-positive, PI double-positive cells—red) 36 h post transfection. Differences compared with mock-transfected cells were calculated using the Mann–Whitney test (* P <0.05). Error bars represent s.d. from four independent transfections. Top error bars relate to Annexin staining, whereas lower error bars represent s.d. for PI staining among Annexin+ cells. DMSO, dimethylsulfoxide; NS, not significant. ( g ) 3DPCR gels after QT6 transfections with A3 constructs along with 5Me-dC-substituted HIV-1 env gene matrix. Asterisks denote the samples that were cloned and sequenced. ( h ) 5′ Dinucleotide analysis of the deamination context performed on minus strand DNA. *Significant deviation from expected values ( χ 2 -test, P <0.05, n =25 for A3A, n =29 for A3Bi7, n =14 forA3Btok, n =21 for A3Blan). Full size image Although 3DPCR is not a quantitative technique, A3A consistently outperformed A3B regarding editing activity ( Fig. 2a , and Supplementary Figs 1a and 2a ), suggesting that in vivo editing by A3A is more efficient than A3B. Given that DSB formation is a macroscopic and quantitative method to assess the efficiency of A3A or A3B editing on nuDNA, γH2AX histone phosphorylation gated on A3-V5-tagged-positive cells was probed 48 h post transfection. Where A3A expression resulted in numerous γH2AX foci in HeLa or QT6 cells, transfection with A3Bi7 or A3Btok consistently failed to make detectable DSBs ( Fig. 2e and Supplementary Fig. 3 ). As DSBs are a direct consequence of A3A-mediated catastrophic mutations on cellular DNA ( Supplementary Fig. 4 ), it is possible that A3B failed to induce the number of mutations required for detectable DSB formation. Nonetheless, A3B activity results in genotoxicity ( Fig. 2 ) and apoptosis just as A3A ( Fig. 2f ) [3] . As orthologous mammalian A3A enzymes are capable of deaminating 5Me-dC residues in ssDNA [31] , 5Me-dC deamination being involved in 5Me-CpG mutation hotspots associated with cancer-related genes [37] was analysed as previously described [6] . Both A3Bi7, A3Btok could edit 5Me-dC-substituted HIV-1 env gene DNA similar to the A3A-positive control compared with A3C used as negative control ( Fig. 2g ). Sequencing of 3DPCR products revealed hypermutated sequences with the same 5′TpC dinucleotide editing preference ( Fig. 2h and Supplementary Fig. 2d,e ). The above findings indicate that A3B is a bona fide mutator of chromosomal DNA, although A3A would appear to be the more powerful of the two in vivo ( Fig 2a,e ). Increased DNA damage from the chimaeric A3A transcript A natural 29.5-kb deletion allele occurs between an identical 370-bp segment spanning intron 4/exon5 of A3A and intron 7/exon8 of A3B. It leaves a chimaeric A3-A3B transcript that differs from normal A3A only by the 3′UTR—the four amino acids of A3A exon 5 and A3B exon 8 being identical ( Fig. 3a and Supplementary Fig. 5 ) [28] . The major difference is the insertion of an Alu sequence in the A3A 3′UTR ( Fig. 3a and Supplementary Fig. 5 ). As previous constructs were C-terminal V5 tagged, a new set of A3A intron 4 constructs were generated, harbouring a N-terminal HA tag and the 3′UTRs from A3A or A3B (UTR A3A and UTR A3B ) ( Fig. 3b ). As can be seen from Fig. 3c transfection of control A3A -ΔUTR, or the chimaeric A3A -UTR A3B construct produced much higher levels of A3A compared with the natural A3A transcript (A3A-UTR A3A ). Reverse transcription quantitative PCR across A3A intron 4 showed a significant twofold reduction in mRNA levels ( Fig. 3d ). To quantify accurately the difference, the UTR sequences were cloned at the 3′ end of the firefly luciferase ( Fig. 3b ) reporter gene and relative luminescence was measured using the Renilla luciferase gene as transfection control. The activity from Luc-ΔUTR and Luc-UTR A3B constructs proved to be ~20-fold greater than that for Luc-UTR A3A ( Fig. 3e ), demonstrating that A3A expression levels of the natural and chimaeric transcripts are primarily controlled by the UTRs. 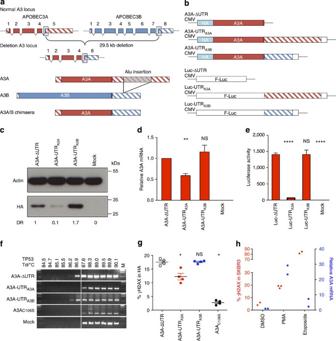Figure 3: A3B deletion locus and enhanced A3A mutation of nuDNA. (a) The A3A–A3B locus and 29.5-kb chimaeric deletion allele along with the three transcripts. (b) A3A-3′UTR and Luc-3′UTR expression constructs cloned into pcDNA3.1 expression vector. (c) Representative western blot analysis from four independent experiments of HA-tagged A3A levels in 293T cells 48 h post transfection with β-actin as loading control. Average expression level is given by densitometric ratio (DR) normalized on actin loading. (d) Transcriptome analysis of the three constructs using oligonucleotides spanning intron 4 and normalized to the expression levels of the housekeeping geneRPL13. Error bars represent s.d. from six independent transfections. Differences compared with Luc-ΔUTR, were calculated using the Mann–Whitney test (**P<0.01). (e) Quantification of UTR-tagged firefly luciferase normalized onRenillaluciferase activity in 293T cells 48 h after transfection. Error bars represent standard deviation from three independent transfections, measured in triplicates. Differences compared to Luc-ΔUTR were calculated using the Mann–Whitney test (****P<0.0001). (f) 3DPCR gel gradients gels for TP53 gene after 293T-UGI transfections with HA-A3 proteins. (g) Fluorescence-activated cell sorting analysis of γH2AX-positive HeLa cells 48 h after transfection gated on the HA-positive cells after A3 transfection. Error bars represent s.d. from four independent transfections. Differences compared with A3A-ΔUTR were calculated using the Mann–Whitney test (*P<0.05). (h) γH2AX-positive DSBs in the ΔA3B−/−cell line SKBR3 treated with 100 μM PMA, 100 μM etoposide and dimethylsulfoxide (DMSO) solvent control (red). Level of endogenous A3A transcript normalized to the expression levels of the housekeeping geneRPL13A(blue). Presented results are from two independent experiments measured in duplicates. NS, not significant. Figure 3: A3B deletion locus and enhanced A3A mutation of nuDNA. ( a ) The A3A–A3B locus and 29.5-kb chimaeric deletion allele along with the three transcripts. ( b ) A3A-3′UTR and Luc-3′UTR expression constructs cloned into pcDNA3.1 expression vector. ( c ) Representative western blot analysis from four independent experiments of HA-tagged A3A levels in 293T cells 48 h post transfection with β-actin as loading control. Average expression level is given by densitometric ratio (DR) normalized on actin loading. ( d ) Transcriptome analysis of the three constructs using oligonucleotides spanning intron 4 and normalized to the expression levels of the housekeeping gene RPL13 . Error bars represent s.d. from six independent transfections. Differences compared with Luc-ΔUTR, were calculated using the Mann–Whitney test (** P <0.01). ( e ) Quantification of UTR-tagged firefly luciferase normalized on Renilla luciferase activity in 293T cells 48 h after transfection. Error bars represent standard deviation from three independent transfections, measured in triplicates. Differences compared to Luc-ΔUTR were calculated using the Mann–Whitney test (**** P <0.0001). ( f ) 3DPCR gel gradients gels for TP53 gene after 293T-UGI transfections with HA-A3 proteins. ( g ) Fluorescence-activated cell sorting analysis of γH2AX-positive HeLa cells 48 h after transfection gated on the HA-positive cells after A3 transfection. Error bars represent s.d. from four independent transfections. Differences compared with A3A-ΔUTR were calculated using the Mann–Whitney test (* P <0.05). ( h ) γH2AX-positive DSBs in the Δ A3B −/− cell line SKBR3 treated with 100 μM PMA, 100 μM etoposide and dimethylsulfoxide (DMSO) solvent control (red). Level of endogenous A3A transcript normalized to the expression levels of the housekeeping gene RPL13A (blue). Presented results are from two independent experiments measured in duplicates. NS, not significant. Full size image To assess A3A cytidine deamination, transfection of 293T-UGI cells showed that the A3A -UTR A3B transcript was capable of hyperediting nuDNA, just as A3A -ΔUTR, while the natural A3A -UTR A3A construct proved to be much less efficient ( Fig. 3f ), a finding paralleled by the frequency of DSBs in HeLa-transfected cells ( Fig. 3g and Supplementary Fig. 6a ). Of note, N-terminal HA-tagged A3A proteins proved somewhat less active than C-terminal V5-tagged constructs ( Fig 3f,g compared with Fig. 2a,e ). The breast cancer cell line SKBR3 harbours the Δ A3B −/− deletion [23] , and sequencing of chimaeric A3A -UTR A3B mRNA transcripts confirmed the deletion between A3A and A3B . As A3A was originally identified following induction by phorbol myristic acetate (PMA) in normal human keratinocytes [38] , SKBR3 cells were treated with 100 μM PMA and DSB formation measured 24 h after induction ( Fig. 3h and Supplementary Fig. 6 ). A3A upregulation was observed in treated SKBR3 cells, accompanied by DSB formation ( Fig. 3h ), confirming that somatic DNA damage can occur in the absence of A3B. Taken together, our results indicate that A3B is an endogenous mutator of nuDNA with dC and 5Me-dC ssDNA substrate specificities, although it seems to access far less efficiently nuDNA than does A3A resulting in modest damage. As established breast cancer-derived cell lines such as HCC1569 and MDA-MB468 express high levels of A3B (ref. 20 ), it would appear that only massive overexpression of A3B leads to experimentally detectable DNA damage. It transpires that the naturally occurring 29.5 kb deletion between a homology region at the 3′ ends of A3A and A3B results in a chimaeric A3A mRNA yielding 10–20-fold higher steady-state levels of A3A leading to increased DNA damage. If a recent study points to lower A3A expression levels among ΔA3B cancers [27] , interpreting tumour-specific A3A and A3B transcription levels needs more work before making correlations with tumour incidence. They can be confounded by the presence of infiltrating haematopoietic cells that generally express much higher levels of A3 genes. A3A levels are generally very low compared with those of A3B , while A3A in effector cells can be massively induced by inflammatory responses [33] , [39] , [40] . In addition, it is not obvious how the accumulation of mutations over a 5–15 or more years are correlated to end-stage tumour A3A and A3B transcription levels. However, as deletion of the entire A3B gene correlates with a higher risk of developing some cancers and an overall higher mutation burden per cancer genome [27] , A3A is clearly an important factor in cancer. As the deletion is associated with a higher odds ratio of developing breast, ovarian and liver cancer, it constitutes a powerful cancer susceptibility marker. These mechanistic findings above tie in well with the recently identified higher mutation burden in breast cancer genomes [27] , indicating that this is causal and not a surrogate marker. They help explain the heterozygous effect between Δ A3B and cancer [24] , [25] , [26] , [27] . Given the sensitivity of A3A to inflammatory environments involving type I and II interferons, while chronic inflammation has long been associated with the onset of cancer [41] , it is distinctly possible that repeated A3A -induced DNA damage will be a major driving force behind iterative somatic mutation/selection of the human genome, cutting across many cancer types. Cancer incidence will be modulated as a function of the global distribution of the Δ A3B polymorphism, with South East Asia where the prevalence of this allele is 35–40% bearing a particularly heavy burden. Plasmids A3B molecular clones were PCR cloned in pcDNA3.1D/V5-His-TOPO vector (Life Technologies). As subcloning of wild-type A3B cDNA into pcDNA3.1D/V5-His-TOPO vector (Life Technologies) proved difficult owing to E. coli toxicity, a synthetic A3B cDNA A3Bi7 containing the 281-bp intron 7 was synthesized (GeneCust) and subsequently cloned in pcDNA3.1D/V5-His-TOPO vector ( Supplementary Table 1 ). Derivatives were then generated by site-directed mutagenesis (GeneArt Site-Directed Mutagenesis System, Life Technologies) ( Supplementary Table 2 ). HA-tagged A3As fused to UTRs were constructed by assembly PCR. A3A-coding sequence retaining the 281-bp intron 4 (GeneCust) was amplified using primers designed to add a N-terminal HA tag, and A3A/A3B 3'UTRs sequences were amplified from 293T genomic DNA extracted using MasterPure complete DNA and RNA purification kit (Epicentre). Overlapping amplicons were purified and mixed for PCR elongation. Full-length constructs were then amplified using external primers ( Supplementary Table 1 ) and cloned in pcDNA3.1D/V5-His-TOPO vector. Luciferase plasmids were constructed the same way using firefly luciferase sequence amplified from pGL4.50[luc2/CMV/Hygro] vector (Promega). All constructs were verified by sequencing. Cells Quail QT6 embryo fibroblast cells were maintained in HAM’s F40 medium (Eurobio), supplemented with 1% chicken serum, 10% FCS, 5% tryptose phosphate, 2 mM L -glutamine, 50 U ml −1 penicillin and 50 mg ml −1 streptomycin. Human HeLa cells, SKBR3 cells and 293T-UGI cells stably expressing Bacillus subtilis phage UGI were maintained in DMEM glutamax medium (Life Technologies) supplemented with 10% FCS, 50 U ml −1 penicillin and 50 mg ml −1 streptomycin. Transfections One million QT6 cells were co-transfected with 0.5 μg of pCayw HBV-coding plasmid and 1.5 μg A3 expression plasmids using JetPrime (Polyplus) following manufacturer’s recommendations and harvested 48 h post transfection. QT6 nuDNA editing was assessed after transfection of 1 μg A3 expression plasmids along with 1 μg of the UGI expression plasmid using the same transfection procedure. For single-plasmid transfections, 8 × 10 5 of HeLa, 293T-UGI, cells were transfected using 2 μg APOBEC3 expression plasmids using JetPrime (Polyplus) following manufacturer’s recommendations and harvested 48 h post transfection. For the 5Me-dC deamination assay, a 679-bp fragment of HIV-1 pNL4.3 env gene was amplified using total substitution of dCTP by 5Me-dCTP (Trilink) using the primer pair 5′-TTGATGATCTGTAGTGCTACAGCA-3′ and 5′-GCCTAATTCCATGTGTACATTGTA-3′. The 5Me-dC containing DNA was heat denatured and chilled on ice, and 200 ng of synthetized DNA was transfected using JetPrime 24 h following initial transfection of APOBEC3-coding plasmids in QT6 cells as described above. For immunofluorescence labelling, 5 10 4 HeLa cells grown on chamber slides (LabTek) were transfected with 1 μg APOBEC3 expression plasmids using Fugene HD (Roche) following manufacturer’s recommendations. For luciferase activity assay, 8 × 10 5 of 293T cells were co-transfected with 1.8 μg of firefly luciferase plasmids along with 0.2 μg of Renilla luciferase control plasmid (Promega). Western blots After blocking, membranes were probed with 1:5,000 diluted mouse monoclonal antibody specific for the V5 epitope (Life Technologies), or 1:2,000 diluted rabbit monoclonal antibody-specific HA tag (Sigma) in PSB (0.01%)–Tween (5%) dry milk applied overnight. After PBS–Tween washings and incubation with an anti-mouse or anti-rabbit IgG horseradish peroxidase-coupled secondary antibody (Amersham), the membrane was revealed by enhanced chemiluminescence (Pierce). β-Actin was used as a loading control using 1:50,000 diluted mouse monoclonal antibody specific for β-actin (Sigma). Signal was quantified using ImageJ software. Uncropped scans of western blots are available in Supplementary Data 1 . Immunofluorescence After PBS washings, transfected HeLa cells grown on chamber slides were fixed with 4% paraformaldehyde for 15 min. After PBS washing, cells were incubated in 50/50 acetone/methanol for 20 min. Mouse monoclonal anti-V5 antibody (Life Technologies) was then incubated at 1:200 for 1 h at room temperature, followed by incubation with 1:500 diluted mouse specific Alexa-488-conjugated goat antibody (Life Technologies) for 1 h at room temperature in the dark. After washing, slides were mounted with Vectashield imaging medium containing 4',6-diamidino-2-phenylindole (Vector Laboratories). Imaging was performed using Leica SP5 confocal microscope. In vitro deamination assay At 72 h post transfection, APOBEC3-transfected 293T cells were extensively washed with PBS and mechanically harvested. Total proteins were extracted using specific lysis buffer (25 mM HEPES (pH 7.4), 10% glycerol, 150 mM NaCl, 0.5% Triton X-100, 1 mM EDTA, 1 mM MgCl 2 and 1 mM ZnCl 2 ) supplemented with protease inhibitors and submitted to sonication. Deaminase activity was assessed by incubating whole-cell lystates with 1 pmol DNA oligonucleotide 5′-(6-FAM)-AAATTCTAATAGATAATGTGA-(TAMRA)-3′ in presence of 0.4 unit uracile-DNA glycosylase (UDG) (NEB) in a 20 mM Tris-HCl, 1 mM dithiothreitol, 1 mM EDTA reaction buffer. After 2 h incubation at 37 °C, generated abasic sites were cleaved by heating 2 min at 95 °C, and end point fluorescence were measured using RealPlex2 Mastercycler (Bio-Rad) with FAM setting and background fluorescence obtained with mock-transfected cells as negative control. Results are normalized to the quantity of protein using Pierce BCA Protein Assay Kit (Thermo Scientific). DNA extraction and 3DPCR amplification Total DNA from transfected cells was extracted using the MasterPure complete DNA and RNA purification kit (Epicentre) and resuspended in 30 μl sterile water. All amplifications were performed using first-round standard PCR followed by nested 3DPCR ( Supplementary Table 3 ). PCR was performed with 1 U Taq DNA polymerase (Eurobio) per reaction. After purification, PCR products were cloned into TOPO 2.1 vector (Life Technologies) and sequencing was outsourced to GATC. Expected values are derived from the base composition of the target sequence assuming no dinucleotide bias (% of NpC=numbers of NpC/numbers of Cs) × 100). Statistical significance of observed percentages compared with expected values was assessed using χ 2 -test. A3A mRNA quantification Transfected 293T cells mRNAs were extracted using RNA EXTRACT RNeasyR Plus Mini Kit (Qiagen). Corresponding cDNAs were synthetized using QuantiTect Reverse Transcription Kit (Qiagen). Quantification was performed by TaqMan using Takyon Rox Probe MasterMix dTTP blue (Eurogentec). A3A mRNA from transfected plasmids was quantified with primers overlapping retained intron4, qA3Afor: 5′-CTGAGGCCCATCCTTCAGTTTCCCT-3′, qA3Arev: 5′-GTGGACCACCAGGGATGT-3′ and molecular probe #11 (Roche). Results were normalized to RPL13A reference gene qRPL13Arev: 5′-CTGGACCGTCTCAAGGTGTT-3′, qRPL13Arev: 5′-GCCCCAGATAGGCAAACTT-3′, probe no. 74. Endogenous level of A3A transcripts in SKBR3 cells was measured a previously described [4] . Luciferase activity Transfected 293T cells (3 × 10 5 ) were split in 96-well plates 24 h after luciferase plasmids transfection. Luciferase activity was measured 24 h later using Dual-Glo luciferase assay (Promega) with 30 min incubation times. Presented results represent luciferase activity from three independent transfections measured in triplicates. Fluorescence-activated cell sorting analysis of apoptosis Transfected HeLa cells were resuspended in binding buffer (BD Pharmingen) and stained with FITC-labelled Annexin V antibody (1 μg ml −1 ; BD Pharmingen). Cells were counterstained 5 μg ml −1 Propidium Iodide (PI) (BD Pharmingen) to distinguish between early apoptotic and late apoptotic or necrotic events. Treatment by 100 μM etoposide in dimethylsulfoxide was used as positive control. Fluorescence-activated cell sorting analysis of DSBs At 48 h after transfection, cells were washed with PBS, fixed in 2–4% ice-cold paraformaldehyde (Electron Microscopy Sciences) for 10 min and permeabilized in 90% ice-cold methanol (Sigma) for 30 min. After washing with PBS, cells were incubated with 1:200 diluted mouse anti-V5 antibody (Life Technologies) in PBS–BSA 0.5% for 1 h. After PBS washings, incubation with 1:500 diluted Alexa Fluor 633 F fragment of goat anti-mouse IgG (H+L) (Life Technologies) was performed for 45 min. HA tag detection was performed in the same conditions using 1:100 anti-HA antibody directly linked to Alexa Fluor 633 (Cell Signaling). DSBs were analysed by staining for 1 h with 1:50 diluted Alexa Fluor 488-conjugated rabbit monoclonal anti-γH2AX (20E3) antibody (Cell Signaling). All incubation steps were performed on ice. Stained samples were acquired on a MACSQuant Analyser (Miltenyi Biotech), and data were analysed with FlowJo software (Tree Star Inc. version 8.7.1). DSB probing in SKBR3 cells was performed 24 h after 100 μM PMA (Sigma) induction with 1:50 diluted Alexa Fluor 647-conjugated rabbit monoclonal anti-γH2AX (20E3) antibody (Cell Signaling). How to cite this article : Caval, V. et al. A prevalent cancer susceptibility APOBEC3A hybrid allele bearing APOBEC3B 3′UTR enhances chromosomal DNA damage. Nat. Commun. 5:5129 doi: 10.1038/ncomms6129 (2014).